Electric-field control of anomalous and topological Hall effects in oxide bilayer thin films One of the key goals in spintronics is to tame the spin-orbit coupling (SOC) that links spin and motion of electrons, giving rise to intriguing magneto-transport properties in itinerant magnets. Prominent examples of such SOC-based phenomena are the anomalous and topological Hall effects. However, controlling them with electric fields has remained unachieved since an electric field tends to be screened in itinerant magnets. Here we demonstrate that both anomalous and topological Hall effects can be modulated by electric fields in oxide heterostructures consisting of ferromagnetic SrRuO 3 and nonmagnetic SrIrO 3 . We observe a clear electric field effect only when SrIrO 3 is inserted between SrRuO 3 and a gate dielectric. Our results establish that strong SOC of nonmagnetic materials such as SrIrO 3 is essential in electrical tuning of these Hall effects and possibly other SOC-related phenomena. Profound implications for the electric field control of spin states have been revealed through magneto-transport properties arising from the spin-orbit coupling (SOC) [1] . Such properties have been attracting great interest as foundations for high-density and low-power-consumption spintronic devices because the properties coupled to the spin states enable spin manipulation without magnetic field variation or large current injection. Among the magneto-transport processes, of interest here is the intrinsic anomalous Hall effect [2] (AHE), which is related to magnetization ( M ) in Hall resistivity ( ρ AHE = R S M ). In some itinerant ferromagnets such as SrRuO 3 [3] , [4] , the proportionality factor ( R S ) is governed by k -space monopoles, i.e., singularities originating from band-crossings gapped by SOC; not M but R S is potentially tuneable by electric field there. Another intriguing example is the topological Hall effect (THE) originating from scalar spin chirality concomitant with non-coplanar spin structures such as in a frustrated pyrochlore magnet [5] and in metallic magnets characterized by a non-zero skyrmion number ( N sk ) [6] , [7] , [8] , [9] . In the case of N sk = 1, the topologically protected spin swirling texture is called magnetic skyrmion [6] , [10] , [11] . Despite mounting interest in electrical control of these Hall effects, however, their control in itinerant magnets has been elusive in conventional field-effect structures, that is, magnetic materials adjacent to gate dielectrics. Recent discovery of the THE in an oxide heterostructure composed of SrRuO 3 and SrIrO 3 [12] brings an opportunity to develop electrical control because the strong SOC in SrIrO 3 [13] induces a SOC-related phenomenon in neighboring ferromagnetic SrRuO 3 . In addition to the intrinsic AHE inherent to SrRuO 3 [3] , the combination of the strong SOC and the broken inversion symmetry gives rise to substantial Dzyaloshinskii–Moriya interaction (DMI) [6] , [14] and the concomitant THE; the underlying spin texture has been deduced to be the interface-driven skyrmion [12] . In view of the fact that ultrathin films of itinerant magnets have been a playground for electrical manipulation of spin states [1] , [15] , [16] , [17] , [18] , [19] , an electric field applied to the ultrathin heterostructure may provoke effective manipulation of the spin state contending with screening effects by itinerant electrons of SrRuO 3 . Furthermore, we can expect that the strong SOC in SrIrO 3 plays a positive role at the interface as well because both AHE and THE are magneto-transport phenomena driven by SOC. Here, we show the clear modulation of both AHE and THE by an electric field in the heterostructure of SrRuO 3 /SrIrO 3 /SrTiO 3 from magneto-transport and magneto-optic Kerr effect (MOKE) measurements. The electrical modulation is effective only when SrIrO 3 is inserted between SrRuO 3 and a gate dielectric, i.e., SrTiO 3 . This indicates the essential role of the strong SOC in nonmagnetic materials for the electrical tuning of these Hall effects and possibly other SOC-related phenomena. Stacking-order dependent electric field control Five-unit-cell SrRuO 3 thin films were epitaxially grown on SrTiO 3 (001) substrates by pulsed laser deposition in three stacking orders with SrIrO 3 (see Methods): a single layer of SrRuO 3 (SRO5/Sub), a bilayer of SrRuO 3 and 2-unit-cell SrIrO 3 (SIO2/SRO5/Sub), and that with the inverted deposition order (SRO5/SIO2/Sub, Fig. 1a ). We first take a look at basic transport and magnetic properties before we go into the Hall effects under an applied electric field (Fig. 1b ). In Fig. 1c, d , we show the temperature dependence of longitudinal resistivity ( ρ xx ) and magnetization perpendicular to the film plane in the three samples. All of them show metallic conduction and ferromagnetic magnetization whose Curie temperatures ( T C ) are lower than the bulk value (160 K) [3] . These transport and magnetic properties are consistent with previously reported ultrathin SrRuO 3 films [20] . 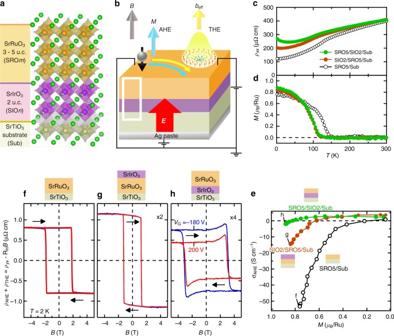Fig. 1 Structure and basic physical properties of samples.aSchematics of the SrRuO3-SrIrO3bilayer film, where SrIrO3is inserted between SrRuO3and SrTiO3substrate (SROm/SIO2/Sub,m= 3–5 unit cells). Green, orange, purple, beige, and gray atoms represent Sr, Ru, Ir, Ti, and O, respectively, in the crystal structure, which is drawn using VESTA38.bSchematics of the magneto-transport properties observed in SROm/SIO2/Sub under the application of a gate electric field (E): Anomalous Hall effect (AHE) generated by magnetization (M) and topological Hall effect (THE) driven by fictitious magnetic field (beff) in the case of skyrmion formation. White box corresponds to the schematics ina. Temperature (T) dependence of longitudinal resistivity (ρxx,c) and out-of-plane magnetization measured at 0.1 T (M,d) for SRO5/Sub, SIO2/SRO5/Sub, and SRO5/SIO2/Sub.eAnomalous Hall conductivity (σAHE) as a function of magnetization (M).f–hThe sum of anomalous and topological Hall resistivity (ρAHE+ρTHE) at 2 K as a function of external magnetic field (B) under application of gate biasVG= − 180 V (blue lines) and 200 V (red lines). At the lowest temperature (T= 2 K), the largest modulation of carrier density can be realized due to the quantum paraelectric nature of SrTiO3substrates. On top, respective sample structure is shown.ρAHE+ρTHEis deduced by subtracting aB-linear ordinary Hall component (RHB) from the Hall resistivity (ρyx). Black arrows indicate the sweep direction ofB Figure 1e shows anomalous Hall conductivity ( σ ΑΗΕ ) as a function of magnetization with temperature as a control parameter. The σ AHE of the three samples behave the same way; when the magnetization gets larger, the sign of σ AHE is inverted from positive to negative. This sign inversion is consistent with the previous experiments [4] , [12] , manifesting the above-mentioned band anti-crossing singularities of SrRuO 3 . Conversely, such temperature dependence in AHE implies the potential for electrical control of AHE through the modification of the SOC-induced band. Fig. 1 Structure and basic physical properties of samples. a Schematics of the SrRuO 3 -SrIrO 3 bilayer film, where SrIrO 3 is inserted between SrRuO 3 and SrTiO 3 substrate (SRO m /SIO2/Sub, m = 3–5 unit cells). Green, orange, purple, beige, and gray atoms represent Sr, Ru, Ir, Ti, and O, respectively, in the crystal structure, which is drawn using VESTA [38] . b Schematics of the magneto-transport properties observed in SRO m /SIO2/Sub under the application of a gate electric field ( E ): Anomalous Hall effect (AHE) generated by magnetization ( M ) and topological Hall effect (THE) driven by fictitious magnetic field ( b eff ) in the case of skyrmion formation. White box corresponds to the schematics in a . Temperature ( T ) dependence of longitudinal resistivity ( ρ xx , c ) and out-of-plane magnetization measured at 0.1 T ( M , d ) for SRO5/Sub, SIO2/SRO5/Sub, and SRO5/SIO2/Sub. e Anomalous Hall conductivity ( σ AHE ) as a function of magnetization ( M ). f – h The sum of anomalous and topological Hall resistivity ( ρ AHE + ρ THE ) at 2 K as a function of external magnetic field ( B ) under application of gate bias V G = − 180 V (blue lines) and 200 V (red lines). At the lowest temperature ( T = 2 K), the largest modulation of carrier density can be realized due to the quantum paraelectric nature of SrTiO 3 substrates. On top, respective sample structure is shown. ρ AHE + ρ THE is deduced by subtracting a B -linear ordinary Hall component ( R H B ) from the Hall resistivity ( ρ yx ). Black arrows indicate the sweep direction of B Full size image In contrast to the similarities of the basic transport and magnetic properties among the three samples, a clear difference emerges in electric field effect (see Methods). The sums of anomalous and topological Hall resistivities ( ρ AHE + ρ THE ) under applied electric fields are shown in Figs. 1f–h as a function of external magnetic field ( B ). The B dependence of ρ AHE corresponds to that of magnetization normal to the film plane, whereas ρ THE shows up with the formation of the topological spin texture as exemplified by the peak at around 3 T in Fig. 1h . The sum of these Hall components is obtained by subtracting the B -linear ordinary Hall term ( R H B ) from the Hall resistivity ( ρ yx ). Both in SRO5/Sub (Fig. 1f ) and in SIO2/SRO5/Sub (Fig. 1g ), ρ AHE + ρ THE is almost unchanged by the applied electric field. However, ρ AHE + ρ THE is obviously changed in SRO5/SIO2/Sub (Fig. 1h ). This striking stacking-order dependence suggests that the electric field to the SrRuO 3 -SrIrO 3 interface causes the noticeable modulation. The thinness of the SrIrO 3 layer compared with the SrRuO 3 layer contributes to the preferable modulation in SRO5/SIO2/Sub because the interface in SRO5/SIO2/Sub is closer to the gate dielectric than that in SIO2/SRO5/Sub (see Supplementary Figure 1 and Supplementary Note 1 ). Hereafter, we focus on the control in the SRO5/SIO2/Sub sample. Electric-field modulation of AHE In the structure of SRO5/SIO2/Sub, the large electric field modulation gives rise to the sign inversion of AHE without changing temperature. Magnetic-field dependences of ρ AHE + ρ THE under different electric fields at 30 K are shown in Fig. 2a–c . Except for the topological Hall term that shows a peak at around 0.8 T, the data are dominated by the anomalous Hall contribution. In particular, we can consider the value at high magnetic field such as 2 T to be totally derived from ρ AHE since all the spins are ferromagnetically aligned without forming any topological spin textures. The sign of ρ AHE above the saturation field is inverted from negative to positive when the gate voltage is varied from negative (−180 V) to positive (200 V), while ρ AHE is close to vanish under zero bias. 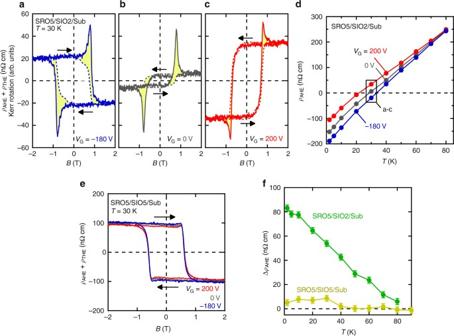Fig. 2 Electric-field control of anomalous Hall effect. Magnetic-field (B) dependence of anomalous and topological Hall resistivities (ρAHE+ρTHE, solid lines) at 30 K under gate voltageVG= −180 V (a), 0 V (b), and 200 V (c) for SRO5/SIO2/Sub. Magneto-optic Kerr rotation as a function ofBunder the same gate bias is also shown by broken lines in each panel. Yellow colored regions correspond toρTHE. Black arrows indicate the sweep direction ofB.dTemperature (T) dependence ofρAHEunderVG= −180 V (blue), 0 V (gray) and 200 V (red). The black box corresponds to the data ina–c.eBdependence ofρAHE+ρTHEat 30 K underVG= −180 V (blue), 0 V (gray), and 200 V (red) for SRO5/SIO5/Sub.fTdependence of variation in anomalous Hall resistivity (ΔρAHE) betweenVG= 200 V andVG= −180 V for SRO5/SIO5/Sub (yellow) and SRO5/SIO2/Sub (green). Error bars include the uncertainty of the sample thickness and of electrical measurement This sign inversion indicates the sign reversal of the proportionality factor R S because MOKE measurements reveal that only a minor fraction of M , <10% of the magnetization, is electrically modulated (see Supplementary Figure 2 and Supplementary Note 2 ). Such electrical sign inversion has never been observed in plain films of itinerant magnets including SrRuO 3 . Fig. 2 Electric-field control of anomalous Hall effect. Magnetic-field ( B ) dependence of anomalous and topological Hall resistivities ( ρ AHE + ρ THE , solid lines) at 30 K under gate voltage V G = −180 V ( a ), 0 V ( b ), and 200 V ( c ) for SRO5/SIO2/Sub. Magneto-optic Kerr rotation as a function of B under the same gate bias is also shown by broken lines in each panel. Yellow colored regions correspond to ρ THE . Black arrows indicate the sweep direction of B . d Temperature ( T ) dependence of ρ AHE under V G = −180 V (blue), 0 V (gray) and 200 V (red). The black box corresponds to the data in a – c . e B dependence of ρ AHE + ρ THE at 30 K under V G = −180 V (blue), 0 V (gray), and 200 V (red) for SRO5/SIO5/Sub. f T dependence of variation in anomalous Hall resistivity (Δ ρ AHE ) between V G = 200 V and V G = −180 V for SRO5/SIO5/Sub (yellow) and SRO5/SIO2/Sub (green). Error bars include the uncertainty of the sample thickness and of electrical measurement Full size image As shown in Fig. 2d , the tendency of AHE change is nearly temperature independent; the positive (negative) bias voltage increases (decreases) ρ AHE regardless of the sign of AHE. Since singularities in the band structure of SrRuO 3 originate from band anti-crossings gapped by SOC, we speculate that the electric field control of AHE is ascribed to the redistribution of the singularities caused by the variation of SOC. The pronounced controllability in SRO5/SIO2/Sub compared with its absence in SIO2/SRO5/Sub suggests that the electric field from SrIrO 3 side induces certain modification of SOC in the bilayer even if it has itinerant carrier density as high as 10 22 cm −3 in the magnetic SrRuO 3 layer. This is in sharp contrast to the case of chemically doped EuTiO 3 [21] , where carrier-density variation inverts the sign of AHE accompanied by the shift of Fermi energy ( E F ). The insertion of the SrIrO 3 layer makes a more important contribution to the AHE modulation than the E F shift in SrRuO 3 does. The controllability may partly rely on the lower carrier density of inserted semimetallic SrIrO 3 , the order of 10 19 cm −3 [22] . In order to clarify the effectiveness of the heterointerface close to the gate dielectric, we also fabricate the heterostructure with thicker (5 unit cells) SrIrO 3 (SRO5/SIO5/Sub, see Supplementary Figures 3 – 5 and Supplementary Notes 3 and 4 ). Figure 2e shows magnetic field dependences of ρ AHE + ρ THE under different electric fields at 30 K in SRO5/SIO5/Sub, where the change of ρ AHE is apparently suppressed. In Fig. 2f , we compare the variation of ρ AHE (Δ ρ AHE = ρ AHE ( V G = 200 V)− ρ AHE ( V G = −180 V)) in SRO5/SIO5/Sub with that in SRO5/SIO2/Sub, where we can clearly see the suppression of the modulation in the thicker SrIrO 3 sample within all the measured temperatures. We attribute this suppression to the significant screening of the electric field within the thicker SrIrO 3 layer. Electric-field modulation of THE THE is also modulated by electric field in the structure of SRO5/SIO2/Sub. In order to evaluate ρ THE from magneto-transport measurement, ρ AHE has to be subtracted from ρ AHE + ρ THE . Since MOKE is proportional to magnetization as anticipated from its perturbative nature and also as experimentally verified in the previous report [12] , MOKE under applied electric field can be utilized as the reference of ρ AHE , which is also proportional to magnetization at a constant temperature. The magnetic field dependences of Kerr rotation are shown by the broken lines in Fig. 2a–c . Each Kerr rotation is normalized by ρ AHE at high magnetic field under each applied electric field; the normalized curves represent the B dependence of ρ AHE . By subtracting them from ρ AHE + ρ THE , we deduced ρ THE (yellow colored regions in Fig. 2a–c ). 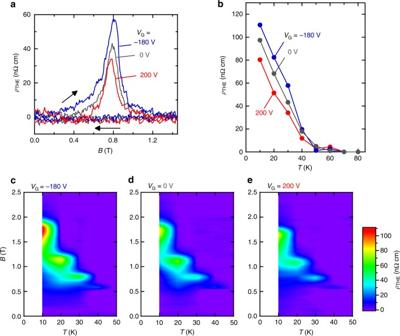Fig. 3 Electric-field control of topological Hall effect.aTopological Hall resistivity (ρTHE) at 30 K as a function of external magnetic field (B) underVG= −180 V (blue line), 0 V (gray line) and 200 V (red line) for SRO5/SIO2/Sub. Black arrows indicate the sweep direction ofB.bTemperature (T) dependence ofρTHEunder gate bias. Color map ofρTHEin theT-Bplane underVG= −180 V (c), 0 V (d) and 200 V (e) 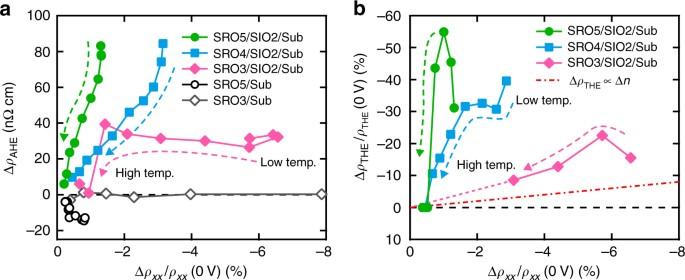Fig. 4 Qualitative analyses of modulations in AHE and THE.aDifference in anomalous Hall resistivity (ΔρAHE) betweenVG= 200 V andVG= −180 V as a function of longitudinal resistivity variation ratio (Δρxx/ρxx(0 V)) at temperatures ranging from 2 K to 80 K.bModulation ratio of topological Hall resistivity (ΔρTHE/ρTHE(0 V)) as a function of Δρxx/ρxx(0 V). Red dash-dotted line is the calculated variation where gate bias only changes carrier density (Δn). Pink dotted line is the guide to the eyes. Broken arrows indicate temperature variation Figure 3a shows the electric field-controlled peak of ρ THE around B = 0.8 T. The electric field also tunes the range of magnetic field where finite ρ THE appears; when the positive (negative) gate voltage is applied, ρ THE gets smaller (larger) and the magnetic field region gets shrunk (enlarged). The variation in peak of ρ THE (Δ ρ THE = ρ THE ( V G = 200 V)− ρ THE ( V G = −180 V)) normalized by zero-bias value (Δ ρ THE / ρ THE (0 V)) is as large as 55%. The sign of THE remains the same during the sign inversion of AHE by electric field, supporting that the origins of AHE and THE are clearly distinct from each other as previously indicated [12] . Fig. 3 Electric-field control of topological Hall effect. a Topological Hall resistivity ( ρ THE ) at 30 K as a function of external magnetic field ( B ) under V G = −180 V (blue line), 0 V (gray line) and 200 V (red line) for SRO5/SIO2/Sub. Black arrows indicate the sweep direction of B . b Temperature ( T ) dependence of ρ THE under gate bias. Color map of ρ THE in the T - B plane under V G = −180 V ( c ), 0 V ( d ) and 200 V ( e ) Full size image Assuming the skyrmion formation in this heterostructure, we discuss the relation of this THE modulation with skyrmion length scale. ρ THE is an outgrowth of ordinary Hall effect under fictitious magnetic field ( b eff ) caused by the non-coplanar spin texture of skyrmion [6] . Since one skyrmion generates one flux quantum ( Φ 0 = h / e ), ρ THE is described as a function of skyrmion density ( n sk ): 
    ρ _THE = PR_Hb_eff = PR_Hn_skΦ _0
 (1) where P is spin polarization of conduction electrons in SrRuO 3 . Ordinary Hall coefficient R H is inversely proportional to carrier density. The change of P or R H is negligible because E F in SrRuO 3 remains almost unchanged judging from the variation of ρ xx as small as the order of 1% as discussed later. Therefore, the modulation of ρ THE indicates the change of n sk . The skyrmion size, estimated by \(r_{{\mathrm{sk}}} \cong 1/\sqrt {n_{{\mathrm{sk}}}}\) , is varied from 15 nm ( V G = 200 V) to 12 nm ( V G = −180 V) adopting P = −9.5% as a typical value of SrRuO 3 [23] and R H evaluated from the B -linear component of Hall resistivity under V G = 0 V at 30 K. Since r sk is proportional to the ratio of ferromagnetic interaction J to DMI D , or J / D [6] , the positive (negative) gate voltage should increase (decrease) J / D . The controlling knob of ρ THE is thought to be D rather than J ; the variation of J is negligible because the applied electric field hardly varies T C , which can be evaluated by a kink structure in ρ xx [3] (see Supplementary Figure 6 and Supplementary Note 5 ). The real-space observation of such electrical control of skyrmion size would be one of the future challenges. We examine the other possibilities of the underlying spin texture. One of the candidates is the conical spin structure, which is topologically trivial and is reported to give rise to THE-like signal [24] . In our case, this can be excluded since the spin structure is dominated by conventional ferromagnetic phase with finite anisotropy as exemplified by open hysteresis loops in magnetization (see Supplementary Figure 2 ). The possibility of non-coplanar spin structures stabilized only under geometrical frustration [5] , [25] can also be excluded because such frustration is apparently absent in our heterostructure. We then focus on a topological spin texture other than skyrmion e.g., biskyrmion or meron, of which topological number ( N sk ) is not unity [9] , [26] , [27] . The emergent fictitious magnetic field can thus be generalized as n topo N sk Φ 0 , where n topo is the density of the topological spin texture. Since N sk is constant inherent in the topological spin structures and hence independent of the gate bias, the electric field modulation of ρ THE is attributed to the modulation of n topo . In order to realize topologically nontrivial spin structures in SrRuO 3 , the interface-driven DMI is required as discussed in the above-mentioned skyrmion case. The ratio of J / D is inversely correlated with n topo for any type of topological spin textures. The consequence therefore remains the same; positive (negative) gate voltage should increase (decrease) J / D . Considering that the variation of DMI is attributed to the modification of SOC at the interface, both modulations of AHE and THE are brought about by the same origin; this appears in the temperature dependence. The tendency of ρ THE change is independent of temperature as shown in Fig. 3b . The expansion of the observable magnetic field region under negative electric field is discerned at every temperature below 40 K (Fig. 3c–e ). These indicate that the obtained modulation of THE is independent of the sign of AHE, which is inverted at 30 K. The temperature independent trend of the electric field effect on THE is in accord with that on AHE (Fig. 2d ), implying the common origin of SOC variation. In fact, the MOKE measurements indicate that the coercive force ( H C ) is shifted from 0.73 T ( V G = 200 V) to 0.76 T ( V G = −180 V) at 30 K (see Supplementary Figure 2 and Supplementary Note 2 ). This shift of H C also supports the modification of SOC because the magnetic anisotropy originates from SOC. The observed modulations of the AHE and THE are not simply explained by the variation of carrier density. In order to show this clearly, the variations of AHE (Δ ρ AHE ) and THE (Δ ρ THE / ρ THE (0 V)) with different thickness of SrRuO 3 films are shown in Fig. 4a, b , respectively, as a function of ρ xx variation normalized by zero-bias value (Δ ρ xx / ρ xx (0 V)) at various temperatures (see Supplementary Figures 7 – 9 and Supplementary Notes 6 – 8 for detailed transport and magnetic properties). Δ ρ xx / ρ xx (0 V) ranges from 1.2% in SRO5/SIO2/Sub to 6.6% in SRO3/SIO2/Sub at 10 K. Since ρ xx is inversely proportional to carrier density ( n ), the order of magnitude is consistent with the expected electron accumulation by a SrTiO 3 -back-gate transistor (Supplementary Note 8 ). Δ ρ AHE in bilayers indicates that the gate-bias control of AHE has the specific tendency regardless of the film thickness. The same plots of SrRuO 3 single layers (SRO m /Sub) are also depicted for comparison. They have negligible change in AHE, while their ρ xx variation is in the same range with that in bilayers with the same SrRuO 3 thickness. As already pointed out, these results demonstrate the importance of inserting the SrIrO 3 layer rather than the E F shift in SrRuO 3 . According to the equation ( 1 ), ρ THE is proportional not only to n sk (or n topo N sk ) but also to R H . We show the calculated variation of ρ THE contributed from R H , i.e., n variation (Δ R H i.e. Δ n = n ( V G = 200 V) − n ( V G = −180 V)) with the red dash-dotted line in Fig. 4b , assuming small Δ n (Δ R H ∝ Δ n / n 2 , i.e., Δ ρ THE ∝ Δ n ) and V G -independent electron mobility. All the modulations in heterostructures are located far above the red dash-dotted line. Therefore, most of the observed Δ ρ THE is attributed to the change in size of the topological spin texture, i.e., DMI. These pronounced modulations of the AHE and THE are both achieved not by carrier-density variation in SrRuO 3 but by modification of SOC at the interface of SrRuO 3 and SrIrO 3 . Fig. 4 Qualitative analyses of modulations in AHE and THE. a Difference in anomalous Hall resistivity (Δ ρ AHE ) between V G = 200 V and V G = −180 V as a function of longitudinal resistivity variation ratio (Δ ρ xx / ρ xx (0 V)) at temperatures ranging from 2 K to 80 K. b Modulation ratio of topological Hall resistivity (Δ ρ THE / ρ THE (0 V)) as a function of Δ ρ xx / ρ xx (0 V). Red dash-dotted line is the calculated variation where gate bias only changes carrier density (Δ n ). Pink dotted line is the guide to the eyes. Broken arrows indicate temperature variation Full size image Recent theoretical calculations [28] , [29] have revealed that the DMI is enormously affected by the singularities in band structures as well as the AHE, although the precise dependencies differ between them. This has been confirmed in itinerant chiral magnets [30] and a semiconducting Dirac electron system [31] . We speculate that our bilayers have some band deformation when applying an electric field to the interface. In both plots in Fig. 4 , thinner SrRuO 3 films exhibit smaller variation in spite of the larger Δ ρ xx / ρ xx (0 V). This thickness dependence is probably attributed to band structure deformation as observed in the thin limit of SrRuO 3 [32] ; the density of states near E F shrinks as SrRuO 3 gets thinner. One of the plausible pathways in the electric field-induced change of SOC is through the interface potential gradient, which is observed as the electrical control of Rashba-type band splitting in a semiconductor quantum well [33] . In contrast to the conventional Rashba systems, however, we have to take into account of the strong SOC of SrIrO 3 , the magnetic properties of SrRuO 3 , and their strong hybridization. Furthermore, since the itinerant-electron systems including SrRuO 3 and SrIrO 3 have complicated distribution of band-anti-crossings in their band structures [22] , [34] , [35] , the quantitative evaluation of the electric field-induced modulation in the heterostructures requires elaborate theoretical investigation. Nevertheless, the present observations clearly indicate that the electric field applied to the thin SrIrO 3 plays the crucial role in SOC at the interface and even brings about the significant modification of magnetic properties in the neighboring itinerant ferromagnet. The method of inserting a thin nonmagnetic material with strong SOC between a ferromagnet and a gate dielectric may be applicable to tuning many intriguing spin-orbit coupled phenomena such as magnetic anisotropy [15] , domain wall motion [36] and the DMI iteself [37] . Sample preparation The epitaxial bilayers composed of SrIrO 3 and SrRuO 3 , and single layer films of SrRuO 3 were deposited on SrTiO 3 (001) substrates by pulsed laser deposition using a KrF excimer laser ( λ = 248 nm). The substrate temperatures during the growth of SrRuO 3 and SrIrO 3 were 730 °C and 600 °C, respectively, where oxygen partial pressure was 120 mTorr. The laser fluence was 1.2 J/cm 2 for SrRuO 3 and 2.6 J/cm 2 for SrIrO 3 . Measurement of magnetic and transport properties The magnetization data were recorded by a SQUID magnetometer with a magnetic field applied perpendicularly to the film plane and along the magnetic easy axis grown on SrTiO 3 (001). Magneto-optic Kerr effect was measured with a laser at 690 nm wavelength in polar geometry by using a photoelastic modulator. Transport properties were measured in Hall bars cut by a diamond wheel saw (1 mm × 2.5 mm) and ultrasonically bonded with Al wires. The applied current was 10 μA, which corresponds to 3.6 × 10 6 A/m 2 for SRO5/SIO2/Sub. Back-gate transistors were fabricated using 0.5-mm-thick SrTiO 3 substrates as a gate dielectric and silver paste as a gate electrode at the opposite side of the deposited films. Antisymmetrizations were performed for both the Hall resistivity and the Kerr rotation angle. Ordinary Hall term was subtracted from the Hall resistivity by linear fitting in a higher magnetic field region. Data availability The data that support the findings of this study are available from the corresponding author upon request.